Camera-based three-dimensional real-time particle tracking at kHz rates and Ångström accuracy Optical and magnetic tweezers are widely employed to probe the mechanics and activity of individual biomolecular complexes. They rely on micrometre-sized particles to detect molecular conformational changes from the particle position. Real-time particle tracking with Ångström accuracy has so far been only achieved using laser detection through photodiodes. Here we demonstrate that camera-based imaging can provide a similar performance for all three dimensions. Particle imaging at kHz rates is combined, with real-time data processing being accelerated by a graphics-processing unit. For particles that are fixed in the sample cell we can detect 3-Å-sized steps that are introduced by cell translations at rates of 10 Hz, while for DNA-tethered particles 5 Å steps at 1 Hz can be resolved. Moreover, 20 particles can be tracked in parallel with comparable accuracy. Our approach provides a simple and robust way for high-resolution tweezer experiments using multiple particles at a time. In the recent years optical and magnetic tweezers have been applied to study a large variety of biological and non-biological microscale systems [1] , [2] , [3] , [4] , [5] , [6] . These techniques allow to exert force on an individual object and to read out simultaneously its conformational change along the force direction. For both force transduction as well as conformational probing, micrometre-sized beads are used. The position of the bead reports the length changes of the system investigated. It was possible to push the limits of the particle-position tracking such that fundamental step sizes of biological motors could be resolved, for example, the 8-nm steps of the cytoskeleton motor kinesin [7] and even single base pair steps (3.4 Å) of DNA-based motors [8] , [9] , [10] . This provides unprecedented insight into smallest conformational changes of biomolecular systems. Such high-resolution measurements have so far only been reported for optical tweezers, where the trapping laser itself is used for displacement detection through quadrant photo diodes or position-sensitive devices [8] , [10] , [11] . The main advantage of the laser-based particle tracking is the excess amount of photons available when typically using trapping powers at the order of 1 W (corresponding to ~10 19 photons per second). Thus, shot noise at the detector is not limiting at the relevant subsecond timescale if the forward scattered light is analysed. This contrasts imaging-based tracking, where the two- or three-dimensional (2D or 3D) position of particles is inferred from camera images [12] , [13] , [14] . Considering an image size of 100 pixels × 100 pixels and a pixel well depth of ~10,000 electrons, only 10 10 photons would be evaluated when tracking at 100-Hz frame rate even for optimal light conditions. In practice, camera-based tracking is indeed severely limited by shot noise and is therefore typically considered as tracking with low spatial and temporal resolution [15] . However, high-resolution camera-based tracking is potentially much simpler to realize and may provide even higher stability. It requires neither a large optical set-up scheme nor highly stable lasers and laser deflection units [10] , [11] . Instead, it relies only on the actual camera combined with standard wide-field illumination. Furthermore, it can easily be adapted to track many particles in parallel [16] , [17] , [18] . Here we intend to push the limits of camera-based particle tracking by maximizing the number of photons evaluated in order to reduce the shot noise limitation. For this we unify different attempts within our real-time particle-tracking scheme. To maximize photon numbers per image we use a large magnification for particle imaging [14] . In order to increase photon numbers per time even further, we perform high-speed imaging using a CMOS camera, for which real-time tracking in 2D at kHz rates has been previously demonstrated [19] , [20] , [21] . Our goal to maxize the imaging throughput requires, however, to cope with the massive amount of data from high-speed imaging as well as the more elaborate 3D position tracking. To this end, we use real-time data processing in a graphics-processing unit (GPU), which was previously employed to speed up post-processing of image packages acquired at >10 kHz [22] . Combining these approaches allows us to resolve base-pair-sized movements of microbeads on a subsecond timescale as well as the parallel tracking of tens of beads at a time. Our real-time data analysis supports long-term data recording at highest temporal and spatial resolution. Furthermore, it allows in situ control and manipulation of tethered objects. Particle-tracking scheme The particle-tracking set-up is based on a homebuilt inverted microscope ( Fig. 1 ) designed for high mechanical stability. The fluidic sample cell contains fixed polystyrene beads that are firmly attached to the bottom of the cell as well as DNA-tethered magnetic beads. A pair of magnets that is placed on a motorized stage above the cell allows the application of pulling forces on the DNA. The sample cell is mounted on a 3D nanopositiong stage to induce well-determined bead displacements through cell translations. Particle images are projected through the microscope objective on a high-speed CMOS camera that allows real-time streaming of images with 1,280 pixels × 1,024 pixels at 500 Hz to the connected computer. When streaming smaller regions of interest (ROIs) instead of the full frame, the maximum rate grows inversely proportional to the number of pixels considered. Tracking of particle positions is carried out either in high-resolution mode-supporting tracking of up to four particles in parallel with high spatial resolution at kHz rates or in multibead mode-supporting tracking of tens of particles with moderate spatial resolution at rates of up to 500 Hz. 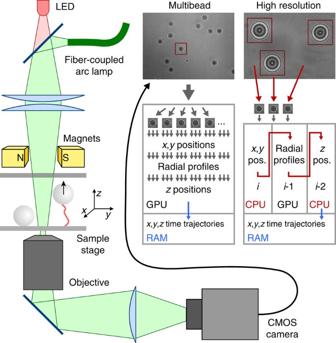Figure 1: Scheme of the particle-tracking set-up and the image analysis routine. Spherical particles within a fluidic cell are mounted on the sample stage of a home-built microscope. The latter comprises a piezo-actuated nanopositiong stage allowing for sample displacements in all three dimensions with Ångström precision. A pair of magnets above the fluidic cell is used to exert forces on DNA-tethered magnetic beads. Tracking of the particle positions is carried out either in high-resolution mode supporting tracking of up to four particles in parallel at high spatial resolution and kHz rates or in multibead mode supporting tracking of tens of particles at moderate spatial resolution and rates up to 500 Hz. For high-resolution tracking, the sample is illuminated using a fibre-coupled mercury lamp. Bead images are acquired simultaneously from distant ROIs using a CMOS camera. Image processing (see red arrows) is carried out in parallel within the CPU regardingx,yandzposition calculations as well as the GPU regarding radial intensity profile calculations. The red squares in the high-resolution sample image indicate the 160 pixels × 160 pixels ROIs that are streamed from the camera into CPU and GPU. For multibead tracking, the sample is illuminated with a 625-nm LED. Full frame images are streamed into the GPU where also all image processing is carried out (see grey arrows). The red square in the multibead sample image corresponds to the size of the 72 pixels × 72 pixels ROIs that are used for tracking. The size of the shown sample image regions is 308 pixels × 224 pixels. Figure 1: Scheme of the particle-tracking set-up and the image analysis routine. Spherical particles within a fluidic cell are mounted on the sample stage of a home-built microscope. The latter comprises a piezo-actuated nanopositiong stage allowing for sample displacements in all three dimensions with Ångström precision. A pair of magnets above the fluidic cell is used to exert forces on DNA-tethered magnetic beads. Tracking of the particle positions is carried out either in high-resolution mode supporting tracking of up to four particles in parallel at high spatial resolution and kHz rates or in multibead mode supporting tracking of tens of particles at moderate spatial resolution and rates up to 500 Hz. For high-resolution tracking, the sample is illuminated using a fibre-coupled mercury lamp. Bead images are acquired simultaneously from distant ROIs using a CMOS camera. Image processing (see red arrows) is carried out in parallel within the CPU regarding x , y and z position calculations as well as the GPU regarding radial intensity profile calculations. The red squares in the high-resolution sample image indicate the 160 pixels × 160 pixels ROIs that are streamed from the camera into CPU and GPU. For multibead tracking, the sample is illuminated with a 625-nm LED. Full frame images are streamed into the GPU where also all image processing is carried out (see grey arrows). The red square in the multibead sample image corresponds to the size of the 72 pixels × 72 pixels ROIs that are used for tracking. The size of the shown sample image regions is 308 pixels × 224 pixels. Full size image For the high-resolution tracking, a large magnification with a conversion factor of 63 nm per pixel is used. Furthermore, we employ the multi-ROI support of the camera and stream up to four independent ROIs of typically 160 pixels × 160 pixels from the camera. The sample is illuminated to fill about half the pixel well depth of the camera. To support tracking rates of up to 3 kHz at the given magnification and achieve a contrast-rich diffraction pattern in the bead images (see below), we use the bright-green emission lines of a fibre-coupled mercury arc lamp. The fibre exit is imaged on the sample by two condenser lenses. Laser or superluminescent diode illumination provides also sufficient light but produces noticeable interference speckles. Therefore, the noncoherent light source was used instead. For image analysis we use a custom-written programme that supports parallel calculations within the computer’s central processing unit (CPU) and the GPU ( Fig. 1 ). The lateral bead positions ( x , y) are determined in the CPU by correlating linear bead intensity profiles with their mirror profiles as described [13] , [20] . Bead images of a single frame are then copied into the GPU where the calculation of the radial intensity distribution with respect to the bead centre is carried out (being the most processing time-consuming step). Images are subdivided into smaller portions to use the high multithreading capability of the GPU. Subsequently, radial intensity profiles are transferred to the CPU to obtain the axial bead position ( z ). This determination uses the diffraction rings of the bead image in overfocus ( Fig. 1 ). The acquired radial profile is compared in an automated manner to a prerecorded profile calibration table [13] , [23] . This table is obtained from imaging the same particle at increasing overfocus values with a step size of typically 25 nm. The three different parts of the tracking routine, that is, image streaming together with lateral position determination, radial intensity calculation and axial position detection, are carried out in parallel. Thus, when the x , y positions of beads from frame i are being calculated in the CPU, the GPU is calculating at the same moment the radial intensity profiles for frame i −1, while additional CPU threads are obtaining the z positions for frame i −2. Although the camera has a built-in dynamic fixed pattern noise (FPN) correction, we used a nonlinear custom-developed FPN correction executed in the GPU. This software-encoded correction further reduces the FPN and avoids artifacts introduced by the dynamic nature of the built-in correction (see Supplementary Fig. 1 ). For each pixel the response–intensity curve is determined and approximated by a three-parameter function that is then used to remove the FPN. This corrects also for the nonlinear pixel response at saturating light levels and inhomogeneous illumination, for example, caused by dirt particles on optical elements along the beam path. Obtained bead positions were stored in memory together with the positions of the magnet and the nanopositioning stage. Bead tracking at kHz rates was thus only limited by the available computer memory and could be carried out continuously for more than 1 h (10 7 frames at 2.5 kHz). For multibead tracking, a lower magnification with a conversion factor of 141 nm per pixel was used to provide a field of view of 180 × 144 μm 2 . The camera was operated in full frame mode at up to 500 Hz. Owing to the six times lower frame rate and the smaller magnification, a standard 625-nm light-emitting diode (LED) provided optimal conditions for sample illumination. LED illumination was preferred here because of the limited life time of the mercury bulb. Streamed images were directly transferred to the GPU, where all the image-processing steps described above were executed. Positions were determined from ROIs of 72 pixels × 72 pixels that comprised the particular bead. Obtained x , y , z positions were transferred every 100 frames to the computer memory μ. Tracking the 3D position of fixed particles We first tested the performance of our high-resolution mode by simultaneously tracking the positions of two 3-μm polystyrene beads that were tightly attached to the bottom of our fluidic cell at 2,500 Hz. When plotting the displacement of the first bead with respect to the second bead (difference coordinate), the measured displacement oscillates around a rather stable mean value with root-mean-square (RMS) values of 1.3 and 1.8 Å for the lateral and the axial positions, respectively ( Fig. 2a ). When smoothing the position trajectories with a sliding average of 10 or 100 ms, the noise is significantly reduced and RMS values down to 0.1 Å are obtained. This suggests that the noise of the bead position determination is largely uncorrelated between successive frames as would be expected for shot noise or white noise in general. 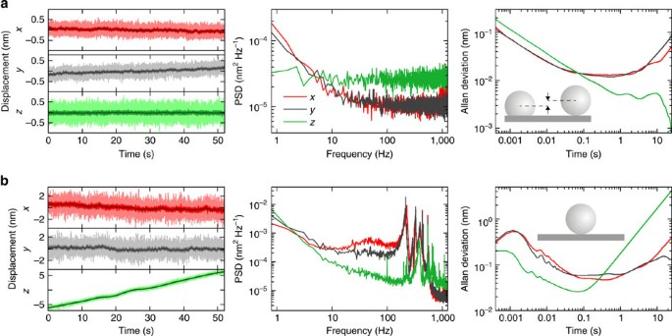Figure 2: 3D tracking of fixed particles. (a) Relative displacement of a 3-μm polystyrene bead bound firmly to the cover glass bottom of the fluidic cell with respect to a second firmly attached reference particle. Shown are time trajectories of the lateral (x,y) and the vertical (z) positions, PSDs and Allan deviations. Position data were taken at 2,500 Hz (light colours) and smoothed to 100 and 10 Hz (intermediate and dark colours, respectively). (b) Displacement of a single bead as function of time from the data set shown ina. Plots and coloring is as ina. Figure 2: 3D tracking of fixed particles. ( a ) Relative displacement of a 3-μm polystyrene bead bound firmly to the cover glass bottom of the fluidic cell with respect to a second firmly attached reference particle. Shown are time trajectories of the lateral ( x , y ) and the vertical ( z ) positions, PSDs and Allan deviations. Position data were taken at 2,500 Hz (light colours) and smoothed to 100 and 10 Hz (intermediate and dark colours, respectively). ( b ) Displacement of a single bead as function of time from the data set shown in a . Plots and coloring is as in a . Full size image To further get insight into the tracking limits, we calculated the power spectral density (PSD) as well as the Allan deviation of the determined trajectories. The PSDs are constant for all coordinates from ~10 Hz, indicating white noise and demonstrating that the positions are uncorrelated for timescales <100 ms. The x and y positions exhibit an increasing PSD for frequencies <10 Hz due to drift, while the axial position seems to be stable even at low frequencies. This behaviour is also seen in the Allan deviations, which is a measure for the position error when smoothing the particle trajectory over a given timescale [24] . For small times τ , the Allan deviation decreases with τ ( − 1/2) confirming uncorrelated noise. For the lateral direction a minimum noise (Allan deviation) of 0.1–0.2 Å is achieved between 100 ms and few seconds. For larger timescales, drift compromises the tracking precision moderately, as can be also seen in the position trajectories. For the axial position, the Allan deviation reaches values significantly below 0.1 Å for τ> 100 ms. These two results demonstrate that we can determine relative position changes of fixed beads with a precision of 1 Å at kHz rates down to 0.1 Å at 10 Hz rates. When plotting the differential position, the second bead serves as a reference that corrects for the drift as well as other noise sources that couple into the microscope set-up. The absolute position of a single particle ( Fig. 2b ) shows consequently increased drift (most prominently along z , see also increasing Allan deviation for times >1 s) as well as an increased RMS amplitude (along x , y ). The latter arises mostly from discrete peaks in the PSDs ( Fig. 2b ) that are absent for the differential positions. Similar peak patterns are also observed in the PSDs calculated from the x , y , z positions of the nanopositioning stage ( Supplementary Fig. 2 ). This indicates that the increased RMS is due to mechanical vibrations that most likely couple in from the laboratory floor or due to sound waves equally affecting both beads. Nonetheless, despite drift and external vibrations, Allan deviations below 1 Å are reached on a timescale of 0.1–1 s for the positions of a single bead ( Fig. 2b ). Resolving 3 Å movements of fixed particles As pointed out above, the Allan deviation characterizes the position error when smoothing the particle trajectory over a given timescale. It is, however, not equal to the minimum resolvable size of sudden steps in the trajectory. Position accuracy (that is, the position error) and resolvable step size are often not stringently distinguished in literature. Typically, only steps amounting to few multiples of the position error at a given timescale can be clearly distinguished [25] . To test whether our set-up is able to resolve base-pair-sized steps, we moved our fluidic cell at fixed time intervals and alternating directions by 3 Å along a given stage direction, while tracking the position of a single bead at 2.5 kHz. We could resolve 3 Å steps of the bead position along all three directions, with a clear correlation between bead and stage position ( Fig. 3 ). For the lateral directions, steps introduced at 1-s intervals could be detected. For the axial direction, steps introduced at 1 s and even 100 ms intervals were discernible, where the higher temporal resolution is due to lower mechanical vibrations of the stage along z . 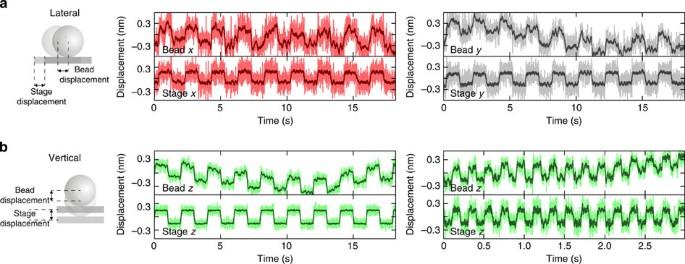Figure 3: Detecting 3-Å steps of fixed particles. (a) Resolving 0.3-nm steps in the lateral direction of a firmly attached 3-μm polystyrene bead. Steps are induced every 1 s by moving the fluidic cell in which the particle is attached with a piezoelectric stage (see sketch). Both, the tracked bead position as well as the simultaneously recorded stage signal are shown over time. (b) Resolving 0.3-nm steps in axial direction that were induced every 1 s or every 100 ms. All data in the figure were recorded at 2,500 Hz. For the 1-s steps the data was smoothed to 100 and 10 Hz (shown as light and dark colours), for the 100 ms steps to 500 Hz (light green) and 100 Hz (dark green). Figure 3: Detecting 3-Å steps of fixed particles. ( a ) Resolving 0.3-nm steps in the lateral direction of a firmly attached 3-μm polystyrene bead. Steps are induced every 1 s by moving the fluidic cell in which the particle is attached with a piezoelectric stage (see sketch). Both, the tracked bead position as well as the simultaneously recorded stage signal are shown over time. ( b ) Resolving 0.3-nm steps in axial direction that were induced every 1 s or every 100 ms. All data in the figure were recorded at 2,500 Hz. For the 1-s steps the data was smoothed to 100 and 10 Hz (shown as light and dark colours), for the 100 ms steps to 500 Hz (light green) and 100 Hz (dark green). Full size image Resolving movements of DNA-tethered particles We next investigated the performance of our particle tracking in a realistic magnetic tweezer configuration. Single 1.9-kbp DNA molecules were attached on one end to the bottom of the fluidic cell and on the other end to a 1-μm magnetic bead. Using a pair of magnets, the DNA was kept stretched under a constant force of 12 pN. The positions of the magnetic bead and of a 3-μm polystyrene bead serving as a reference were tracked simultaneously at 2.8 kHz in high-resolution mode. When plotting the position of the magnetic bead with respect to the reference bead the RMS amplitude is significantly increased in all directions because of the thermal fluctuations of the DNA-tethered bead ( Fig. 4a ). The PSDs in the lateral directions exhibit characteristic Lorentzian shapes, since the pendulum motion of the bead is highly over damped. The restoring force in the pendulum configuration is proportional to the magnetic force. It can be experimentally determined from fitting the characteristic shape of the PSD or alternatively the Allan deviation [26] . Along the axial direction the entropic and the elastic rigidity of DNA determines the extent of the fluctuations [14] , which are at the applied force considerably smaller than in the lateral direction (see trajectories and PSD levels in Fig. 4a ). The Allan deviation reaches a minimum of ~1 Å between 0.1 and 1 s, suggesting that (sub)-nanometre-sized DNA-length changes are detectable. Indeed, when moving the fluidic cell in axial direction in alternating 1 nm steps at 1 s intervals the position changes can be clearly resolved in the magnetic bead position ( Fig. 4b ). When measuring the DNA length the noticeable drift of the magnetic bead position is corrected by the fixed reference particle that exhibits a similar drift. Even 5 Å steps introduced at 1-s intervals are discernible in the magnetic bead position, although less pronounced than for the larger steps ( Fig. 4b ). 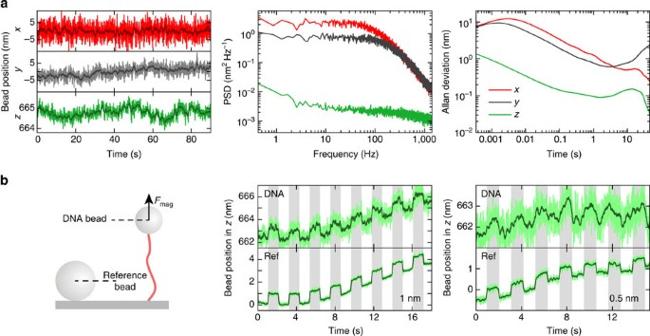Figure 4: Length measurement of a DNA molecule under constant tension. (a) Positions of a 1-μm magnetic bead tethered to a 1.9-kbp DNA molecule under an applied force of 12 pN. Shown are time trajectories of the relative displacements of the bead to an immobilized 3-μm reference bead and the corresponding PSDs and Allan deviations. Position data were taken at 2,800 Hz and smoothed to 10 and 1 Hz (light and dark colours, respectively). (b) Resolving 1 and 0.5 nm steps of a DNA-tethered magnetic bead (as ina) along the vertical direction. Steps in alternating direction were induced about once per second. Positions of the DNA tethered as well as of a fixed reference particle (see sketch) are shown as indicated in the plots. Position data were taken at 2,800 Hz and smoothed to 100 and 10 Hz (shown in light and dark green, respectively). Figure 4: Length measurement of a DNA molecule under constant tension. ( a ) Positions of a 1-μm magnetic bead tethered to a 1.9-kbp DNA molecule under an applied force of 12 pN. Shown are time trajectories of the relative displacements of the bead to an immobilized 3-μm reference bead and the corresponding PSDs and Allan deviations. Position data were taken at 2,800 Hz and smoothed to 10 and 1 Hz (light and dark colours, respectively). ( b ) Resolving 1 and 0.5 nm steps of a DNA-tethered magnetic bead (as in a ) along the vertical direction. Steps in alternating direction were induced about once per second. Positions of the DNA tethered as well as of a fixed reference particle (see sketch) are shown as indicated in the plots. Position data were taken at 2,800 Hz and smoothed to 100 and 10 Hz (shown in light and dark green, respectively). Full size image When looking at the DNA length trajectory and its Allan deviation (differential position of magnetic bead in axial direction in Fig. 4a ) it becomes apparent that for longer timescales the measurement accuracy is not limited by the Brownian motion of the particle but rather by a low-frequency drift component. This component prevents the resolution of sudden steps better than 5 Å. We can rule out that the drift arises from thermal drift of the objective focus with respect to the beads, since it is not reduced when keeping the reference bead at a fixed absolute position through a feedback. We further tested whether the low-frequency drift occurs because of the usage of differently sized beads. The determined position may depend on the actual position in a slightly nonlinear manner, being more pronounced for the smaller magnetic beads. However, when tracking the position of a firmly attached 1-μm magnetic bead versus a firmly attached 3-μm polystyrene reference bead, no relative drift component was apparent (see Supplementary Fig. 3a ). The RMS amplitude of the raw position signal was two- to threefold larger compared with the difference coordinate of two 3-μm beads. Nonetheless, Allan deviations that were significantly lower than 1 Å were still obtained for all coordinates. In addition, 0.3-nm step-wise movements of the fluidic cell in both lateral and vertical directions could be clearly resolved in the magnetic bead position (see Supplementary Fig. 3b,c ). This demonstrates that smaller, 1-μm-sized beads support high-resolution tracking with bp resolution. We therefore attribute the observed low-frequency drift for DNA-tethered beads to instabilities of the magnetic bead orientation [27] , that is, a nanoscale drift in bead alignment with the magnetic field. Highly parallel particle tracking at 3Å resolution We next tested the parallel position tracking of 26 fixed polystyrene beads (3 μm diameter) in multibead mode at a rate of 420 Hz, at which simple LED illumination is sufficient (see above). Steps of 3 Å introduced at 1-s intervals can be resolved in lateral and axial directions for all beads (see trajectories in Fig. 5a,c for three of the beads). The high resolution even in the multibead mode is supported by the Allan deviations of the differential positions with respect to a reference bead ( Fig. 5b,d ). The Allan deviations for different beads are all very similar reaching values significantly below 1 Å from ~0.1 s onwards. 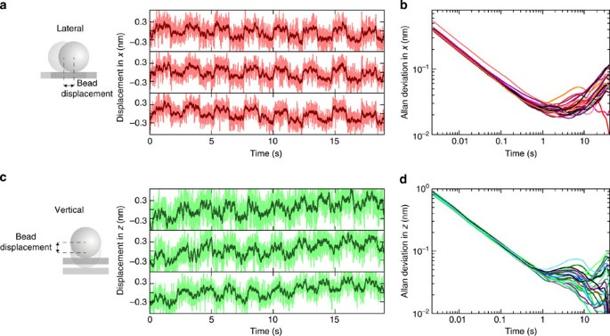Figure 5: Parallel tracking of multiple beads with subnanometre resolution. The 3D positions of 26 firmly attached 3-μm polystyrene beads were tracked simultaneously at 420 Hz. (a) Example of time traces of three of the 26 beads in which the piezoelectric stage was moved every 1 s by 0.3 nm in alternating direction along thexaxis (see sketch). Shown position data were smoothed to 105 and 10 Hz (shown as light and dark red). (b) Allan deviations of the relative positions of all 26 beads against a reference bead in the lateral direction. (c) Example of time traces of three of the 26 beads in which the piezoelectric stage was moved every 1 s by 0.3 nm in alternating direction along thezaxis (see sketch). Shown position data were smoothed to 105 and 10 Hz (shown as light and dark green). (d) Allan deviations of the relative positions of all 26 beads against a reference bead in the vertical direction. Figure 5: Parallel tracking of multiple beads with subnanometre resolution. The 3D positions of 26 firmly attached 3-μm polystyrene beads were tracked simultaneously at 420 Hz. ( a ) Example of time traces of three of the 26 beads in which the piezoelectric stage was moved every 1 s by 0.3 nm in alternating direction along the x axis (see sketch). Shown position data were smoothed to 105 and 10 Hz (shown as light and dark red). ( b ) Allan deviations of the relative positions of all 26 beads against a reference bead in the lateral direction. ( c ) Example of time traces of three of the 26 beads in which the piezoelectric stage was moved every 1 s by 0.3 nm in alternating direction along the z axis (see sketch). Shown position data were smoothed to 105 and 10 Hz (shown as light and dark green). ( d ) Allan deviations of the relative positions of all 26 beads against a reference bead in the vertical direction. Full size image Here we introduce a real-time particle-tracking scheme capable of resolving base-pair-sized movements of particles on a (sub-)second timescale. We thus obtain a similar sensitivity as high-resolution optical tweezers with laser-based detection [11] , despite a much simpler set-up design. For laser-based detection, only one or two beads can be tracked at a time with high resolution. Here we exploit the potential of camera-based tracking and demonstrate that we can resolve base-pair-sized steps in a highly parallel manner on tens of beads simultaneously at only little compromised tracking accuracy. When tracking two particles in parallel at highest spatial resolution (per frame taken), we obtain rates of up to 3 kHz (corresponding to processing of 150 MB s −1 of image data). Thus, our tracking scheme can also be applied to resolve fast dynamics of biomolecular systems at millisecond timescales and subnanometre spatial resolution. Compared with rates in laser tracking of up to MHz, our camera-based tracking is still dynamically limited. The frame transfer from the camera to the computer would at least allow for approximately fourfold faster image acquisition. However, currently the computational power of CPU and GPU as well as the availability of noncoherent light sources with sufficient brightness do not permit faster tracking at comparable accuracy. Nonetheless, in the range of milliseconds to seconds, which is most often the timescale of interest for biomolecular systems, similar or even better spatial accuracies as for laser tracking are achieved. Previous camera-based tracking approaches reached rates of >10 kHz for 2D real-time tracking [20] and 3D tracking with image postprocessing [22] . The larger rates were obtained at the expense of lower magnifications and thus much lower numbers of pixels per bead image. Taking more pixels per image of the same physical size provides a higher tracking accuracy per frame (compare Allan deviations at lowest times in Figs 2 and 5 ) [18] . In addition, it greatly reduces position bias due to pixilation effects [28] (the dependence of the obtained bead position on the actual bead position with respect to the pixel lattice) and thus also drift. As a result, the Allan deviations obtained here are at comparable timescales significantly lower than in previous reports. The GPU-supported high-resolution real-time particle tracking presented here was applied within a regular magnetic tweezer scheme for which 3D position information is mandatory. It is based on previously established tracking methodology and can therefore be easily adapted for existing instruments. Accomplishing real-time tracking at kHz rates allows to cope with the massive image data being produced. This conveniently supports continuous long-term measurements with high spatiotemporal resolution but also in situ manipulation of objects, as typically carried out in tweezer measurements. Previous high-resolution magnetic tweezers applied image post processing, which limited the continuous acquisition to ~10 s (ref. 22 ). Beyond achieving base-pair accuracy for camera-based magnetic and optical tweezer systems, our particle-tracking scheme will also provide a considerable improvement for particle-tracking applications that need to handle large image sets. This includes highly parallelized experiments in multiplexed holographic optical tweezers [19] , multiplexed magnetic tweezers with up to 10 3 simultaneous measurements [17] , multiplexed particle experiments in liquid flow [29] or fast real-time particle velocimetry [30] . Currently, the particle positions in these applications are typically obtained not in real-time but rather from stored image data only after each measurement. Our real-time particle-tracking scheme will not only allow for experiments with extended duration and thus better statistics but by using larger camera chips even more particles per experiment can be followed with higher accuracy. Given that we can analyse 26 particles at 420 Hz, it will be equally possible to follow ~200 particles at 60 Hz. Thus, our approach will greatly simplify highly parallel measurements of enzymatic activity [16] , [29] and facilitate the detection of rare events. In addition, for single-molecule DNA-sequencing applications relying on mechanical force detection [31] our high-throughput real-time tracking promises significant improvements over current state-of-the-art technology. Furthermore, the outsourcing of the image processing to the GPU is ideally suited for experiments where camera-based real-time particle tracking is combined with simultaneously operating detection channels that require additional computational resources, such as in single-molecule torque measurements [32] , [33] or in set-ups that combine tweezer experiments with single-molecule fluorescence methods [34] , [35] , [36] . When detecting length changes on single DNA molecules, the presented magnetic tweezers data do not yet reach single-base-pair resolution but rather 5–10 Å. As explained above, we believe that this limitation stems from imperfections of the magnetic particles. With improved magnetic particles that possess a more stable anisotropy axis the mentioned problems may be overcome. Therefore, with the high tracking accuracy presented here and because of the stable and simple set-up design, routine magnetic tweezers measurements on DNA with single-base-pair resolution should be achievable. Particle-tracking set-up The particle-tracking set-up consisted of a home-built inverted microscope body equipped with either a × 100 (Olympus, N.A. 1.25) or a 40 × (Zeiss, N.A. 1.3) oil immersion objective for high-resolution or multibead tracking modes, respectively. The bead sample is mounted on a piezo-actuated nanopositioning stage (P-517.3CD, PI). The sample was illuminated using either a fibre-coupled mercury arc lamp (LSB610, LOT-Oriel) equipped with a 550/100-nm band pass filter (AHF Analysentechnik) or an LED emitting at ~625 nm (CR5111AWY, Roithner Lasertechnik). Both light sources were combined using a 605-nm dichroic mirror (AHF Analysentechnik). Bead images were projected through a 400-mm tube lens on a high-speed CMOS camera (Mikrotron EoSens CL MC1362). Two permanent NeFeB magnets (W-05-N50-G, Supermagnete) mounted on a motorized stage above the sample were used to generate the magnetic field gradient for the magnetic tweezers experiments. A data acquisition card (USB-6281M, National Instruments) was used to record the signals from the nanopositioning stage in a synchronized manner. A trigger pulse from the camera at the beginning of a frame acquisition was used to generate a pulse train of 10 rectangular pulses during the frame acquisition time. The subpulses then triggered the acquisition of the stage positions. The 10 readouts were averaged to obtain a mean stage position per frame with reduced read noise. Data (images, stage positions) were streamed to a computer (Dell precision T7500 work station containing two 6-core CPUs) equipped with an image acquisition card (NI PCIe 1429, National Instruments) and a fast GPU (GeForce GTX 480, Nvidia). Set-up control as well as data acquisition and processing were carried out by a custom-developed software (Labview 2010 64-bit version, National Instruments). GPU programming was carried out in CUDA C and compiled as a dynamic-link library (DLL) for embedding into Labview. An implementation of our software supporting offline tracking can be downloaded from the author’s webpage. Tracking experiments Fluidic cells were built from two cover slides and a parafilm spacer that formed the final chamber. The bottom cover slip was spin-coated on the inside with polystyrene before cell assembly. The cell was mounted on the set-up using a custom-designed plate on the nanopositioning stage. Carboxylated polystyrene beads (3 μm; Invitrogen) in 1 M NaCl were added and incubated for at least 1 h to ensure adherence to the polystyrene film. Subsequently, PBS was added for the measurements with fixed beads. Magnetic tweezers experiments with DNA-tethered beads were carried out [14] using a 1.9-kbp DNA molecule carrying at either end a 600-bp DNA fragment with multiple digoxigenin or biotin modifications as previously described [37] . In brief, after adhering the fixed beads, the fluidic cell was incubated with 50 μg ml −l anti-digoxigenin in PBS for 1 h. Afterwards, it was incubated for 1 h with 10 mg ml −1 BSA to prevent nonspecific binding to the bottom of the cell. The DNA construct was bound to 1 μm magnetic beads in PBS and added to the fluidic cell. After 5 min, non-tethered beads were removed by approaching the magnets and subsequent buffer flushing. Subsequently, sets of calibration profiles were recorded for appropriate beads and tracking experiments were started. For the experiments with fixed 1 μm magnetic beads ( Supplementary Fig. 3 ), both magnetic and reference beads were adhered to bare (uncoated) cover slides. After sample-drying, the slide was placed for 3 min on a hot plate at 150 °C to allow bead fixation as described [22] . Afterwards, the fluidic cell was assembled and PBS was added in order to carry out the tracking measurements. Data analysis Smoothing of shown trajectories was carried out using a sliding average with the indicated window size. PSDs were calculated from long trajectories that were split into 40 equally long parts. PSDs of these subtrajectories were averaged to provide the PSDs shown. Allan deviations were calculated from overlapping time intervals using a computationally efficient form [26] , [38] . How to cite this article: Huhle, A. et al . Camera-based three-dimensional real-time particle tracking at kHz rates and Ångström accuracy. Nat. Commun. 6:5885 doi: 10.1038/ncomms6885 (2015).